Somatic transcriptome priming gates lineage-specific differentiation potential of human-induced pluripotent stem cell states Human-induced pluripotent stem cells (hiPSCs) provide an invaluable source for regenerative medicine, but are limited by proficient lineage-specific differentiation. Here we reveal that hiPSCs derived from human fibroblasts (Fibs) versus human cord blood (CB) exhibit indistinguishable pluripotency, but harbour biased propensities for differentiation. Genes associated with germ layer specification were identical in Fib- or CB-derived iPSCs, whereas lineage-specific marks emerge upon differentiation induction of hiPSCs that were correlated to the cell of origin. Differentiation propensities come at the expense of other lineages and cannot be overcome with stimuli for alternative cell fates. Although incomplete DNA methylation and distinct histone modifications of lineage-specific loci correlate to lineage-specific transcriptome priming, transitioning hiPSCs into naive state of pluripotency removes iPSC-memorized transcriptome. Upon re-entry to the primed state, transcriptome memory is restored, indicating a human-specific phenomenon whereby lineage gated developmental potential is not permanently erased, but can be modulated by the pluripotent state. Expression of a discrete and defined set of gene products associated with pluripotency (OCT4, SOX2, c-MYC, KLF4, NANOG and LIN28) induces reprogramming of somatic cells into self-renewing pluripotent cell types similar to human embryonic stem cells (ESCs) [1] , [2] . While morphology, pluripotent gene expression profiles and pluripotent markers in human-induced pluripotent stem cells (hiPSCs) are suggestive of equipotent developmental potential, recent studies reveal substantial molecular and functional differences among iPSCs derived from distinct cell types. iPSCs produced different properties in teratoma formation that correlate with the tissue of origin [3] and moreover, persistence of the DNA methylation status of the cell of origin has been linked with molecular aspects of hiPSC programming [4] . Aside from these molecular descriptions, transcriptome analysis and functional measurements, such as lineage-specific maturation potential have yet to be robustly examined. Recently, iPSCs have been shown to retain a DNA methylation status akin to the cell of origin [4] , [5] , [6] , [7] . However, to date, no causal evidence has been presented to suggest that incomplete methylation is responsible for imposing memory, as opposed to a consequence of unknown mechanisms, which drive the observed changes in epigenetic status of specific loci or whether this impacts differentiation behaviour. One of the most promising applications of iPSCs is to model human disease, and is only limited by efficient and controlled differentiation of human PSCs into specific cell types. Here we generated hiPSCs from different sources, adult dermal fibroblasts (Fibs) and CD34 + umbilical cord blood (CB) cells, and functionally and quantitatively compared their differentiation potential along with transcriptional profiles in the undifferentiated state. Cell fate decisions were shown to closely relate to the transcriptional profiles connected to lineage of origin, and did not extend to the corresponding germ layer. We propose that the differentiation potential of human iPSCs is channelled towards the parental lineage, but this comes at the expense of differentiation to other cell types. Equivalency of pluripotent states of hiPSCs Molecular and functional properties of human hiPSCs derived from different somatic sources were compared between hiPSCs generated from CD34 + CD45 + umbilical CB cells and compared with iPSCs from human adult dermal Fibs, a common source for iPSC generation. Inclusion of CD45 was critical to assure cells used were of a hematopoietic lineage, and not endothelial cells that also express CD34 (refs 8 , 9 ). To provide generalizable results, all hiPSC lines were derived by transduction with Oct4 , Sox2 , Nanog and Lin28 or Oct4 , Sox2 , c-Myc and KIf4 expressing lentiviral vectors. Both hFib and hCB-derived iPSC lines were morphologically indistinguishable from hESCs and acquired typical pluripotent marker expression, similar among hiPSCs and hESCs ( Fig. 1a ). Both hFib- and hCB-iPSCs exhibited comparable transcript levels of the genes associated with pluripotency ( Dppa4 , Tbx3 , c-Myc , Oct4 , Sox2 and Nanog ), similar to hESCs ( Supplementary Fig. 1a,b ) and produced teratomas containing the three embryonic germ layers ( Fig. 1b ). Moreover, global gene expression profiling followed by hierarchical cluster analysis on genes associated with pluripotency further indicated successful molecular reprogramming to the pluripotent state ( Fig. 1c ). Clustering of hiPSCs lines with hESCs by principal component analysis, and no significant differences between hFib- versus hCB-iPSCs in gene set-enrichment analysis (GSEA) provided additional evidence that Fib- and CB-iPSCs are not distinguishable by evaluating pluripotent status ( Supplementary Fig. 1c,d ). Collectively, these results indicate that using molecular and functional criteria routinely applied to characterize fully reprogrammed iPSCs, hCB-iPSCs and hFib-iPSCs are indistinguishable using established criteria for the human pluripotent state [2] , [10] . 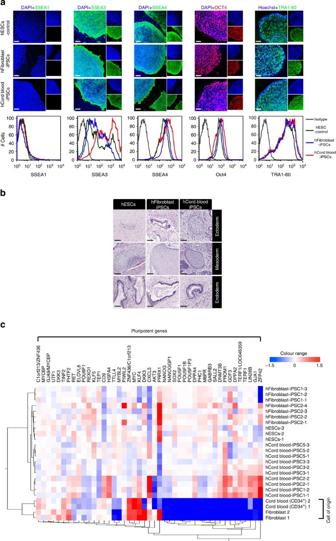Figure 1: Equivalency of pluripotent states of hiPSCs derived from cord blood and fibroblasts. (a) Immunocytochemical analysis for pluripotent markers SSEA-1, SSEA-3, SSEA-4, OCT4 and TRA-1-60 in hESCs, fibroblast- and cord blood-iPSCs. Nuclei are stained with DAPI or Hoechst 33342. At the bottom is shown representative flow cytometry analysis for pluripotent markers SSEA-1, SSEA-3, SSEA-4, OCT4 and TRA-1-60. Scale bars, 100 μm. (b) Teratomas production by hESC and hiPSC lines. Haematoxylin–eosin-stained sections show differentiation into all three germ layers: ectoderm, endoderm and mesoderm. Scale bars, 200 μm. (c) Hierarchical cluster analysis using genes associated with pluripotency. Dendrogram branch lengths are based on Pearson’s correlation coefficients. Each row represents a gene. Figure 1: Equivalency of pluripotent states of hiPSCs derived from cord blood and fibroblasts. ( a ) Immunocytochemical analysis for pluripotent markers SSEA-1, SSEA-3, SSEA-4, OCT4 and TRA-1-60 in hESCs, fibroblast- and cord blood-iPSCs. Nuclei are stained with DAPI or Hoechst 33342. At the bottom is shown representative flow cytometry analysis for pluripotent markers SSEA-1, SSEA-3, SSEA-4, OCT4 and TRA-1-60. Scale bars, 100 μm. ( b ) Teratomas production by hESC and hiPSC lines. Haematoxylin–eosin-stained sections show differentiation into all three germ layers: ectoderm, endoderm and mesoderm. Scale bars, 200 μm. ( c ) Hierarchical cluster analysis using genes associated with pluripotency. Dendrogram branch lengths are based on Pearson’s correlation coefficients. Each row represents a gene. Full size image Equivalency in transcriptional profiles of three germ layers Recent reports indicate that incomplete DNA methylation underlies transcriptional differences in iPSCs derived from different origins/tissues, suggesting that cellular memory persists in the iPSCs following reprogramming [4] , and that this phenomenon is unique to human iPSCs as mouse iPSCs lose this memory over passaging [5] . To better understand whether previously observed differential propensities for one lineage versus another followed a developmental paradigm (for example, could lineage augmentation be due to an initial increased overall germ layer propensity), we analysed gene expression patterns corresponding to the three germ layers (ectoderm, endoderm and mesoderm). Hierarchical clustering on genes related to ectoderm, endoderm and mesoderm emergence revealed similar patterns across all PSCs from all cell sources, methods and clones of human iPSCs ( Fig. 2a,d,g ). Furthermore, we directly compared germ layer-related expression between hCB- and hFib-iPSCs through GSEA, which revealed no significant differences between hiPSC lines ( Fig. 2b,e,h ), suggesting that somatic memory cannot be explained by inherent activation of transcription related to the specification stage of germ layer commitment within the pluripotent state. As such, we next examined whether the apparent discrepancy in the differentiation capacity of hiPSCs from different somatic origins was due to a disparity in the initiation of early developmental programmes related to lineage-specific commitment. To assess this, we initiated differentiation in hiPSCs towards specific lineages, neural (ectoderm), hepatocytes (endoderm), cardiomyocytes and hematopoietic (mesoderm), and examined early lineage-associated markers. Early neural marker, PAX6 ( Fig. 2c ), and hematopoietic markers, brachyury (T) and MixL1 ( Fig. 2i ), showed marked differences in the initial stage of differentiation, wherein hCB-iPSCs displayed increased hematopoietic and decreased neural marker expression compared with hFib-iPSCs ( Fig. 2c,i ). However, no clear expression differences were observed between hCB- and hFib-iPSCs for endodermal markers, FoxA2, Gata4 and Sox17 ( Fig. 2f ; Supplementary Fig. 2 ), or the mesodermal marker smooth muscle actin (SMA) ( Fig. 2i ) during early developmental progression into hepatocytic and cardiomyocytic lineages, respectively. This indicates that hiPSCs possess a biased lineage specification towards cell types closely related to the tissue of origin. Overall, these results reveal that pre-existing germ layer transcriptional activity is equivalent in hiPSCs, but lineage-specific transcription becomes gradually unbalanced in a stepwise manner during early-induced commitment stages of hPSC development. 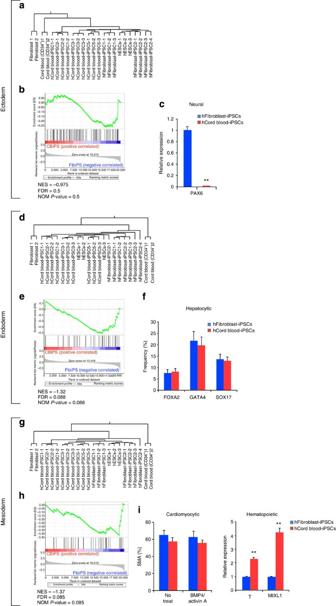Figure 2: Equivalency in transcriptional profiles of three germ layers. (a) Hierarchical cluster analysis using genes associated with ectoderm lineage. (b) GSEA plot of enrichment of gene signature related to ectoderm lineage between fibroblast- versus cord blood-iPSCs. (c) Quantitative RT-PCR analysis of early neural marker,PAX6. Samples are purified at day 4 during neural differentiation. Individual reactions were normalized according to GAPDH. (n=6). (d) Hierarchical cluster analysis with genes of endoderm lineage. (e) GSEA plot of enrichment of gene signature associated with endoderm lineage between fibroblast- versus cord blood-iPSCs. (f) Frequency of FOXA2-, GATA4- and SOX17-positive cells for endoderm formation during hepatocyte generation (n=14). (g) Hierarchical cluster analysis with genes of mesoderm lineage. (h) GSEA plot of enrichment of gene signature related to mesoderm lineage. (i) (left) Percentage of smooth muscle actin (SMA)-positive cells at day 7 during cardiomyocyte differentiation, performed in hEBs medium supplemented with activating factors (BMP4 and Activin A) or not (n=5). (Right) quantitative RT-PCR analysis for mesodermal markers,MixL1andBrachyury (T), during hematopoietic differentiation (day 4). Individual reactions were normalized according to GAPDH. (n=6). All data are represented as mean±s.e.m. **P<0.01, Student’st-test. Figure 2: Equivalency in transcriptional profiles of three germ layers. ( a ) Hierarchical cluster analysis using genes associated with ectoderm lineage. ( b ) GSEA plot of enrichment of gene signature related to ectoderm lineage between fibroblast- versus cord blood-iPSCs. ( c ) Quantitative RT-PCR analysis of early neural marker, PAX6 . Samples are purified at day 4 during neural differentiation. Individual reactions were normalized according to GAPDH. ( n =6). ( d ) Hierarchical cluster analysis with genes of endoderm lineage. ( e ) GSEA plot of enrichment of gene signature associated with endoderm lineage between fibroblast- versus cord blood-iPSCs. ( f ) Frequency of FOXA2-, GATA4- and SOX17-positive cells for endoderm formation during hepatocyte generation ( n =14). ( g ) Hierarchical cluster analysis with genes of mesoderm lineage. ( h ) GSEA plot of enrichment of gene signature related to mesoderm lineage. ( i ) (left) Percentage of smooth muscle actin (SMA)-positive cells at day 7 during cardiomyocyte differentiation, performed in hEBs medium supplemented with activating factors (BMP4 and Activin A) or not ( n =5). (Right) quantitative RT-PCR analysis for mesodermal markers, MixL1 and Brachyury (T) , during hematopoietic differentiation (day 4). Individual reactions were normalized according to GAPDH. ( n =6). All data are represented as mean±s.e.m. ** P <0.01, Student’s t -test. Full size image Distinct differentiation potential in hFib- versus hCB-iPSCs To functionally assess the consequence of differential activation of lineage-specific transcription between hiPSCs from different cellular origins, we further evaluated their in vitro differentiation potential starting with neural lineage specification. Neural lineage differentiation was evaluated in two stages; the initial analysis encompassed formation of neural precursor/progenitors followed by differentiation into the three major cell types found in the central nervous system: neurons, oligodendrocytes and astrocytes [11] , [12] . Neurospheres, representing an early neural progenitor/precursor stage, were generated from dissociated hiPSCs, expanded and then differentiated using previously optimized protocols [11] , [12] . In contrast to the comparable gene expression of ectodermal lineage markers in undifferentiated cells, hCB-iPSCs produced significantly less neural precursor/progenitor cells after neural differentiation induction ( Fig. 3a ). hCB-iPSC-derived precurser/progenitors were significantly less proliferative during neurosphere-forming assays and displayed fewer nestin- and A2B5-positive cells compared with Fib-iPSCs ( Fig. 3b,c ). In accordance with these differential outcomes of neural differentiation, analyses of neural-specific gene expression in undifferentiated hCB- and hFib-iPSCs revealed significantly downregulated expression of NF68 and NEUROD1 in cells derived from CB compared with Fibs, further strengthening the correlation between phenotypic outcome and lineage-specific transcriptional control ( Fig. 3d ). 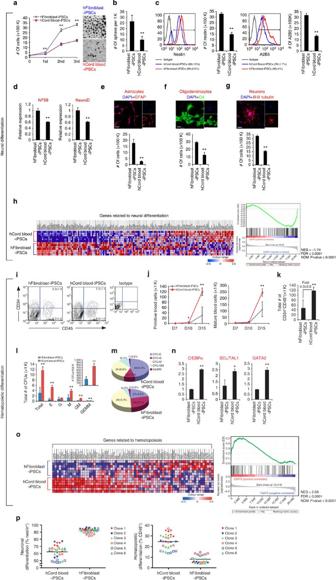Figure 3: Distinct differentiation potential in hiPSCs derived from fibroblasts and cord blood. (a) Quantitative results of neurosphere expansion (n=14). Right panel shows the images of neurosphere generated at the end of the 2nd expansion cycle of hiPSCs. Scale bars, 200 μm. (b) Quantification of the neurosphere generation capacity from 1 K numbers of cells (n=18). (c) Representative flow cytometry plots for neural stem cell marker nestin and the neural precursor marker A2B5 in neurosphere. Right panel shows total number of nestin- or A2B5-positive cells. (n=10). (d) Quantitative RT-PCR analysis of neural-specific genes from undifferentiated cells. Individual reactions were normalized to GAPDH. (n=6). Neural stem cells from hiPSCs were further differentiated into astrocytes as indicted by GFAP staining (e, top panel), oligodendrocytes as indicated by O4 staining (f, top panel) and neurons as indicated by β-III-tubulin staining (g, top panel). Scale bars, 50 μm (e,f) and 100 μm (g). Bottom panels fore–gare graphs for quantification of total number of differentiated cells of respective neural lineages (n=10). (h) GSEA plot of gene signatures related to neural lineage (right) and heat map of genes (left). (i) Representative fluorescence-activated cell sorting plot for the expression of primitive blood cells markers, CD34 and CD45, of hiPSCs hEBs after 15 days hEB culture. (j) Total number of differentiated primitive blood cells and mature blood cells in hEBs from hiPSCs over days 7, 10 and 15 (n=14). (k) Total number of differentiated CD34+CD45+cells from hiPSCs (n=10). (l) Total number of hematopoietic CFUs and number of colony subtypes generated from day 15 hEBs. Inset shows hematopoietic progenitor capacity of hEBs. (n=10). (m) Distribution of colony subtypes derived from hiPSC lines. (n) Quantitative RT-PCR analysis for blood-specific genes. Samples are purified from undifferentiated cells and individual reactions were normalized to GAPDH. (n=6). (o) GSEA plot of enrichment of gene signature related to hematopoietic lineage (right) and heat map of genes (left). (p) Quantification of expression of neural stem cell marker nestin during neural differentiation (left). Quantitative results of CD45+-positive cells during hematopoietic differentiation (right). All bars indicate average of all clones. All data are represented as mean±s.e.m. *P<0.05, **P<0.01, Student’st-test. Figure 3: Distinct differentiation potential in hiPSCs derived from fibroblasts and cord blood. ( a ) Quantitative results of neurosphere expansion ( n =14). Right panel shows the images of neurosphere generated at the end of the 2nd expansion cycle of hiPSCs. Scale bars, 200 μm. ( b ) Quantification of the neurosphere generation capacity from 1 K numbers of cells ( n =18). ( c ) Representative flow cytometry plots for neural stem cell marker nestin and the neural precursor marker A2B5 in neurosphere. Right panel shows total number of nestin- or A2B5-positive cells. ( n =10). ( d ) Quantitative RT-PCR analysis of neural-specific genes from undifferentiated cells. Individual reactions were normalized to GAPDH. ( n =6). Neural stem cells from hiPSCs were further differentiated into astrocytes as indicted by GFAP staining ( e , top panel), oligodendrocytes as indicated by O4 staining ( f , top panel) and neurons as indicated by β-III-tubulin staining ( g , top panel). Scale bars, 50 μm ( e , f ) and 100 μm ( g ). Bottom panels for e – g are graphs for quantification of total number of differentiated cells of respective neural lineages ( n =10). ( h ) GSEA plot of gene signatures related to neural lineage (right) and heat map of genes (left). ( i ) Representative fluorescence-activated cell sorting plot for the expression of primitive blood cells markers, CD34 and CD45, of hiPSCs hEBs after 15 days hEB culture. ( j ) Total number of differentiated primitive blood cells and mature blood cells in hEBs from hiPSCs over days 7, 10 and 15 ( n =14). ( k ) Total number of differentiated CD34 + CD45 + cells from hiPSCs ( n =10). ( l ) Total number of hematopoietic CFUs and number of colony subtypes generated from day 15 hEBs. Inset shows hematopoietic progenitor capacity of hEBs. ( n =10). ( m ) Distribution of colony subtypes derived from hiPSC lines. ( n ) Quantitative RT-PCR analysis for blood-specific genes. Samples are purified from undifferentiated cells and individual reactions were normalized to GAPDH. ( n =6). ( o ) GSEA plot of enrichment of gene signature related to hematopoietic lineage (right) and heat map of genes (left). ( p ) Quantification of expression of neural stem cell marker nestin during neural differentiation (left). Quantitative results of CD45 + -positive cells during hematopoietic differentiation (right). All bars indicate average of all clones. All data are represented as mean±s.e.m. * P <0.05, ** P <0.01, Student’s t -test. Full size image Neural precursors from both CB- and Fib-iPSCs were further differentiated into neurons, oligodendrocytes and astrocytes [11] , [12] . While both hiPSC lines were capable of generating all three neural cell types, quantitative analysis revealed that the reduced ability of hCB-iPSCs to produce neural progenitor cells translated into a reduced number of GFAP-, O4- and βIII-Tubulin-positive cells representative of astrocytes, oligodendrocytes and neurons, respectively ( Fig. 3e–g ). These results suggest that differentiation towards the neural lineage is limited in hCB-iPSCs, but this limitation does not affect the resulting progenitor differentiation potential. To evaluate whether this limitation in differentiation potential was transcriptionally encoded in the undifferentiated state, we performed GSEA using a neural lineage gene set ( Fig. 3h , right panel) between hCB- and hFib-iPSCs ( Fig. 3h , left panel). While gene expression profiles of ectodermal development were comparable between hiPSCs ( Fig. 2b ), neural gene expression in hCB-iPSCs was significantly inhibited ( Fig. 3h ), indicating that biological differentiation outcomes are likely controlled by lineage-specific programming (not germ layer specification) within pluripotent cells. To better understand predetermined cell fate decisions of undifferentiated hiPSCs, we broadened our comparison to evaluate in vitro hematopoietic differentiation, which represents the parental lineage of hCB-iPSCs. Human embryoid bodies (hEBs) were generated from cell lines of both Fib and blood origin, and the frequency of cells expressing hematopoietic markers was assessed [13] . Following hEB formation, an increase in the frequency of primitive blood (CD34 + CD45 + ) cells was observed in hCB-iPSCs when compared with hFib-iPSCs ( Fig. 3i ). Marked generation of primitive (CD34 + CD45 + ) and mature (CD34 - CD45 + ) blood cells also demonstrated an augmented response of hCB-hiPSCs to hematopoietic-specific signals ( Fig. 3j ). As a consequence, the overall number of hematopoietic cells generated was highly enriched from hCB-iPSCs ( Fig. 3k ). To further compare the multi-lineage potential of hiPSC-derived hematopoietic progenitors from different cell origins, we performed hematopoietic colony-forming unit (CFU) assays ( Supplementary Fig. 3a ). In line with increased generation of CD34 + CD45 + cells, hCB-iPSCs produced more CFUs than hFib-iPSCs ( Fig. 3l ), indicating that enhanced acquisition of the hematopoietic phenotype does not occur at the expense of progenitor function. Analysis of specific hematopoietic developmental potential revealed biased differentiation of progenitors derived from hCB-iPSCs into CFU-erythroid (CFU-E), while the frequency of CFU-macrophage (CFU-M) and CFU-granulocyte (CFU-G) was lower compared with hFib-iPSCs ( Fig. 3m ). Having confirmed the expected hematopoietic differentiation bias of hiPSCs derived from CB, we next analysed undifferentiated hCB-iPSCs for transcriptional activity related to hematopoietic programmes. In line with the correlation between downregulated neural gene expression and poor neural differentiation, hCB-iPSCs displayed higher expression levels of critical hematopoiesis genes such as, C/EBPα , Scl/Tal and GATA2 (ref. 14 ), compared with hFib-iPSCs ( Fig. 3n ), demonstrating that hCB-iPSCs are predisposed towards the hematopoietic fate. Moreover, GSEA of genes associated with the hematopoietic lineage [15] , [16] revealed a highly enriched hematopoietic signature in hCB-iPSCs, further supporting that differentiation potential is transcriptionally encoded in the undifferentiated state ( Fig. 3o ). To validate the observed differentiation disparities present in hCB- and hFib-iPSCs, we analysed multiple clones from three independent CB and two independent Fib donors that were reprogrammed with two distinct methodologies for both neural and hematopoietic differentiation. Each individual clone clearly revealed biased differentiation propensity of hFib- versus hCB-iPSCs towards neural versus hematopoietic fates, respectively ( Fig. 3p ), suggesting that cellular origin affects differentiation propensity of hiPSCs regardless of reprogramming factors or the donor sample used ( Supplementary Table 3 ). Moreover, unlike murine iPSC memory that is erased after 10 passages, this disparity in differentiation potential was not altered by prolonged culture examined (20 passages) ( Supplementary Fig. 3b,c ), implying sustained functional discrepancy among hiPSCs, in contrast to mouse iPSCs [4] , [6] . Predetermined decision of hCB-iPSCs into hematopoietic lineage To further evaluate the basis of maintained somatic lineage preferences in hFib- versus hCB-iPSCs, we expanded our analysis to other mesodermal cell types in addition to hematopoietic differentiation, such as cardiomyocyte development. In contrast to hematopoietic differentiation capacity, cardiomyocytic fate was limited in hCB-iPSCs, even in the presence of activating growth and inducing factors ( Supplementary Fig. 4a ). While both hiPSC lines were capable of generating comparable frequencies of the smooth muscle marker SMA ( Fig. 2i ), the expression of the mature cardiomyocyte markers, including isoform of Troponin T (cTnT), was markedly reduced in hCB-iPSCs ( Supplementary Fig. 4b,c ). Compared with GSEA of hematopoietic genes, hCB-iPSCs displayed reduced expression of genes associated with cardiomyocytic fates ( Supplementary Fig. 4d ), highlighting that the differentiation propensity of pluripotent cells is governed by the underlying somatic transcriptome associated with the cell of origin. Since differentiation potential is highly correlative to the transcriptional profiles related to the cellular origin of established hiPSCs, we generated hEBs in the absence of exogenous stimuli conductive to a specific lineage to explore whether spontaneous differentiation can be affected by the inherent transcriptome distinctions among hiPSCs. Although the overall number of hematopoietic cells is reduced when compared with cells treated with cytokines ( Fig. 3k ), the relative expansion of primitive blood cells derived from hCB-iPSCs compared with hFib-iPSCs was increased fivefold ( Fig. 4a ). Furthermore, irrespective of the complete absence of hematopoietic factors in vitro , functional capacity of hCB-iPSCs to generate hematopoietic progenitors (CFUs) was higher as compared with hFib-iPSC-derived cells ( Fig. 4a ), suggesting that the hematopoietic lineage propensity is independent of hematopoietic stimuli and is cell autonomous. In addition, hCB-iPSCs preferentially differentiate into the erythroid sub-lineage (CFU-E), compared with hFib-iPSCs ( Fig. 4b ). Overall, these data support that hCB-iPSCs possess enhanced hematopoietic differentiation potential that is predetermined, where the addition of exogenous hematopoietic factors can further augment blood development in hCB-iPSCs. In addition, our results reveal that differentiation potential of hCB-iPSCs is highly tuned towards the cell of origin, while the cardiomyocytic fate of shared germ layer origin is severely compromised. 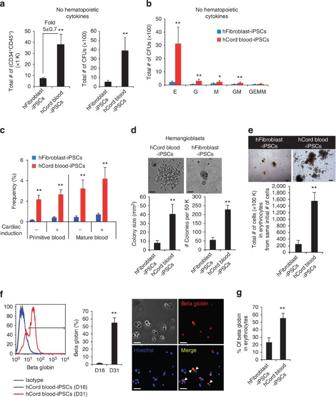Figure 4: Predetermined fate decision of hCB-iPSCs into hematopoietic lineage. (a) Total number of differentiated CD34+CD45+cells from hiPSCs in the absence of hematopoietic cytokines. Number indicates fold change between hiPSCs (left). Total number of hematopoietic CFUs generated from day 15 hEBs without activating factors (right). (n=8). (b) Total number of colony subtypes generated from day 15 hEBs without hematopoietic cytokines (n=6). (c) Maintenance of hematopoietic potentials in hCB-iPSCs under stimuli for alternative cell fates. Frequency of differentiated primitive blood cells and mature blood cells during cardiomyocyte differentiation (n=6). (d) Different size of haemangioblasts colony and colony numbers produced from different hiPSCs. (Top) is phase contrast images showing haemangioblasts derived from hiPSCs. Scale bars, 100 μm. (Bottom) quantification of haemangioblasts sizes and colony numbers (n=12). (e) Quantification of total number of differentiated erythroid cells from hiPSCs-haemangioblast cells (n=9). (Top) representative images of differentiated erythroid cells from hiPSCs. Scale bars, 200 μm. (f) Representative fluorescence-activated cell sorting plot of β-globin expression in erythorid cells at day 16 and day 31 of differentiation and maturation cultures. (Middle) is quantification of flow cytometry (n=9). (Right) is immunostaining of mature erythroid cells, derived from hUCB-iPSCs, with β-globin chain-specific antibody. Nuclei are stained with DAPI. (▸) indicates β-globin-positive and DAPI-negative cells. Scale bars, 50 μm. (g) Quantification of adult β-globin-positive red blood cells from hiPSCs (n=6). All data are represented as mean±s.e.m. *P<0.05, **P<0.01, Student’st-test. Figure 4: Predetermined fate decision of hCB-iPSCs into hematopoietic lineage. ( a ) Total number of differentiated CD34 + CD45 + cells from hiPSCs in the absence of hematopoietic cytokines. Number indicates fold change between hiPSCs (left). Total number of hematopoietic CFUs generated from day 15 hEBs without activating factors (right). ( n =8). ( b ) Total number of colony subtypes generated from day 15 hEBs without hematopoietic cytokines ( n =6). ( c ) Maintenance of hematopoietic potentials in hCB-iPSCs under stimuli for alternative cell fates. Frequency of differentiated primitive blood cells and mature blood cells during cardiomyocyte differentiation ( n =6). ( d ) Different size of haemangioblasts colony and colony numbers produced from different hiPSCs. (Top) is phase contrast images showing haemangioblasts derived from hiPSCs. Scale bars, 100 μm. (Bottom) quantification of haemangioblasts sizes and colony numbers ( n =12). ( e ) Quantification of total number of differentiated erythroid cells from hiPSCs-haemangioblast cells ( n =9). (Top) representative images of differentiated erythroid cells from hiPSCs. Scale bars, 200 μm. ( f ) Representative fluorescence-activated cell sorting plot of β-globin expression in erythorid cells at day 16 and day 31 of differentiation and maturation cultures. (Middle) is quantification of flow cytometry ( n =9). (Right) is immunostaining of mature erythroid cells, derived from hUCB-iPSCs, with β-globin chain-specific antibody. Nuclei are stained with DAPI. ( ▸ ) indicates β-globin-positive and DAPI-negative cells. Scale bars, 50 μm. ( g ) Quantification of adult β-globin-positive red blood cells from hiPSCs ( n =6). All data are represented as mean±s.e.m. * P <0.05, ** P <0.01, Student’s t -test. Full size image On the basis of lineage propensities within a germ layer, we next explored whether hematopoietic differentiation predominates in hCB-iPSCs even under stimuli for alternative cell fates. Marked generation of primitive and mature blood cells during cardiomyocyte conducive differentiation suggest that differentiation of hiPSCs is gated to the specific somatic cell fate associated with their cellular origin, and in doing so restricts alternative cell fates ( Fig. 4c ). Given that CB-hiPSCs retained the donor cell-specific molecular profiles even under stimuli for alternative cell fates, we examined whether those features can be applied for generation of hematopoietic cells with definitive/adult hematopoietic programmes that have been elusive from hPSCs at the functional protein level [17] without stimulation of novel pathways [18] . Recently, an efficient method has been developed to generate large numbers of bipotential progenitors, known as haemangioblasts, which retain both hematopoietic and endothelial potential [19] , [20] . As predicted from previous reports, hiPSC lines could produce haemangioblasts that further differentiated into both endothelial and hematopoietic lineages ( Supplementary Fig. 5a ). Consistently, hCB-iPSCs produced not only a larger number of haemangioblast colonies, but the clonal capacity measured by cellularity was greater compared with hFib-iPSC lines ( Fig. 4d ). In addition, hCB-iPSC-derived haemangioblasts generated more CFUs that preferentially differentiate into CFU-E ( Supplementary Fig. 5b,c ). Although haemangioblasts derived from hCB-iPSCs maintained endohematopoietic differentiation potential, these cells appear biased towards hematopoietic lineages. Giving the overwhelming evidence that progenitors of hCB-iPSCs preferentially differentiate into CFU-E ( Fig. 3m ; Supplementary Fig. 5c ), we further examined erythrocyte generation [21] . Increased numbers of cells were obtained from hCB-iPSCs compared with hFib-iPSCs despite the same number of input haemangioblast cells ( Fig. 4e ). The expression of high levels of glycophorin A (CD235a) and the lack of CD45 on the surface confirmed the presence of erythrocytic features ( Supplementary Fig. 5d ). Further maturation of hCB-iPSC-derived erythrocytes induced a definitive hematopoietic programme as indicated by human adult β-globin protein expression and enucleated erythroid cells ( Fig. 4f,g ), hence hCB-iPSCs show enhanced erythropoiesis differentiation capacity. Taken together, these results demonstrate superior potential of hCB-iPSCs to generate adult β-globin-positive red blood cells, providing insight for targeting explicit somatic cell sources for hiPSC generation intended for lineage-specific applications. Differentially encoded differentiation potential in hiPSCs Recently, we revealed that cell fate potential is encoded within cells comprising hESCs [22] . By marking cells expressing c-KIT (hematopoietic primed) and A2B5 (neural primed), we successfully subfractionated hESCs and demonstrated clear propensities for hematopoietic and neural lineage differentiation, respectively [22] . A significant increase in the frequency of c-KIT-positive cells and reduced A2B5-expressing cells were observed in hCB-iPSCs ( Fig. 5a ), which correlates with increased hematopoietic and reduced neural lineage capacity shown (Fig. 3), thereby supporting the notion that cell fate decisions are differentially predisposed within cells comprising hiPSCs from different somatic sources. To aid in determining the molecular basis of this lineage priming effect, we investigated whether distinct epigenetic modifications of key lineage-specific regulatory genes correlated with lineage propensity demonstrated. Similar to previous reports showing epigenetic memory relates to incomplete DNA methylation, we found distinct methylation status in lineage-related genes, whereas hCB-iPSCs showed decreased methylation in the hematopoietic marker, T ( Fig. 5b ), and increased methylation in the neural marker, PAX6 ( Fig. 5c ), compared with hFib-iPSCs. Moving beyond the methylation status, we investigated for evidence of distinct histone modifications in lineage-specific gene loci for both neural and hematopoietic regulatory genes. hCB-iPSCs displayed enrichment of H3K4me3 activation marks on MIXL1 ( Fig. 5b ) and H3K27me3 repressive marks on NF68 ( Fig. 5c ), further strengthening the current hypothesis of epigenetic regulation that governs distinct differentiation potentials. 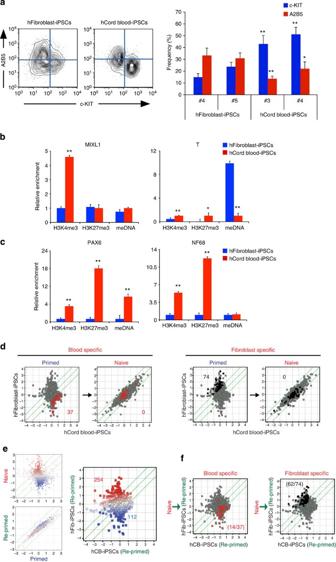Figure 5: Differentially encoded cell differentiation potential in hiPSCs derived from human adult dermal fibroblast and CD34+umbilical cord blood cells. (a) Flow cytometry analysis of the expression of c-KIT and A2B5, associated with mesoderm progenitors and neural precursors, respectively, in undifferentiated hiPSCs. (Right) is percentages of c-KIT- and A2B5-positive cells in hiPSCs (n=5). (b,c) Single ChIP analysis of histone modification and DNA methylation on mesodermal lineage genes (b; T and MIXL1) and neural lineages genes (c; PAX6 and NF68) loci. (n=3). (d) Loss of transcriptional somatic memory in naive conditions. Blood-specific (red) and fibroblast-specific (blue) genes are indicated in global gene expression comparison. (e,f) Conversion into original primed conditions reacquires initial transcriptional differences. All data are represented as mean±s.e.m. *P<0.05, **P<0.01, Student’st-test. Figure 5: Differentially encoded cell differentiation potential in hiPSCs derived from human adult dermal fibroblast and CD34 + umbilical cord blood cells. ( a ) Flow cytometry analysis of the expression of c-KIT and A2B5, associated with mesoderm progenitors and neural precursors, respectively, in undifferentiated hiPSCs. (Right) is percentages of c-KIT- and A2B5-positive cells in hiPSCs ( n =5). ( b , c ) Single ChIP analysis of histone modification and DNA methylation on mesodermal lineage genes ( b ; T and MIXL1) and neural lineages genes ( c ; PAX6 and NF68) loci. ( n =3). ( d ) Loss of transcriptional somatic memory in naive conditions. Blood-specific (red) and fibroblast-specific (blue) genes are indicated in global gene expression comparison. ( e , f ) Conversion into original primed conditions reacquires initial transcriptional differences. All data are represented as mean±s.e.m. * P <0.05, ** P <0.01, Student’s t -test. Full size image Despite displaying similar levels of pluripotent hallmark genes and germ layer specification-related transcriptional programmes, hiPSCs from different somatic sources retain a level of lineage-specific gene activation that results in efficient differentiation towards their cell of origin. Given that murine iPSCs are able to erase this transcriptional memory after serial passaging, yet human cells do not, it is likely that distinct molecular mechanisms are at play in the human scenario. Alternatively, murine and human PSCs rely on different signalling pathways to sustain self-renewal in the pluripotent state, and are cultured in completely different conditions from previous studies comparing iPSC memory; it is possible the ‘state’ of iPSCs (primed versus naive) is critical to memory status. Recent studies have demonstrated that human iPSCs normally considered to be in ‘primed pluripotent state’ can be converted into cells having mouse ESC-like traits, called the ‘naive pluripotent state’ [23] , [24] , [25] . As such, we transitioned our CB- and Fib-derived hiPSCs into the naive PSC state and performed comparative transcriptome analysis. Human iPSCs in the primed state maintain gene expression of their cell of origin, but surprisingly, under naive conditions, hiPSCs rewire and erase transcriptional memory of somatic cells ( Fig. 5d ). In contrast to transcriptional retention of the somatic cell of origin of hiPSCs in the primed state, regardless of cellular origin, similar transcriptional profiles were displayed once hiPSCs were placed in naive state. However, when reversed from the naive state, back to primed conditions, hiPSCs reacquire transcriptional profiles similar to parental hiPSCs and surprisingly, re-established transcriptome memory ( Fig. 5e,f ), implicating the pluripotent ‘state’ as a direct effector of somatic memory for the first time. Efficient and controlled differentiation to specific lineages represents the major barrier for future clinical applications of hiPSCs, including cell replacement therapies and drug discovery [26] . Therefore, a deeper understanding of the starting populations of hiPSCs is required to instruct proficient differentiation. Our study demonstrates that although the hiPSC lines express pluripotent genes and support differentiation into cell types of all three germ layers, measured by established assays for pluripotency [27] , hiPSC lines possess unique functional properties when induced to differentiate, where these distinct properties are predetermined at the transcriptome level of undifferentiated hiPSC states. We propose that although human iPSCs are molecularly and functionally defined as pluripotent, hiPSCs are heterogeneous in their developmental potential and are better defined by ‘lineage gated’ capacity for pluripotency based on cellular origins used to derive hiPSCs. This suggests that determination and characterization of somatic cells for reprogramming may provide enhanced differentiation for specific research and therapeutic applications, and could be tailored accordingly. Mechanistically, it has previously been reported that iPSCs retain DNA methylation profiles of the tissue from which they were derived [5] , [6] , [7] as an explanation for iPSC memory. Our current study supports these findings and further implicates epigenetic modification of histone status as markers of cellular memory within reprogrammed pluripotent cells. However, like DNA methylation, whether these histone modifications are causal determinants or a consequence of additional processes not defined in this study still remain to be elucidated. Beyond these uncertainties, our results reveal that hiPSCs preferentially activate transcriptional programmes related to the specific cell of origin from whence they were derived at the expense of other unrelated lineages. As current differentiation procedures are principally based on desired germ layer targeting, followed by lineages within that germ layer, this suggests that new procedures for hiPSCs that arise from different cells of origin may be unique. Moreover, we now show that like hESCs, cell fate potential is encoded within cells comprising hiPSCs. Phenotypic assessment of newly created iPSC lines for fate-coding markers such as c-KIT and A2B5 could help to provide insight into retained somatic memory and eventual differentiation outcome. Consistent differentiation propensity in the extended passage suggests persistent preservation of molecular and cellular properties in hiPSCs unlike their mouse counterparts, where serial passaging attenuates their differences [4] , [6] . So far, epigenetic memory (incomplete DNA methylation) is the most plausible molecular explanation for somatic memory both of mouse and human iPSCs, but fails to reconcile the causal differences between regulation of mouse and human memory. Our study proposes that the difference in human versus mouse memory is related to primed versus naive states of pluripotency. We have demonstrated that human naive culture conditions rewire and erase transcriptional memory of somatic cells retained in hCB-iPSCs, implicating, for the first time, that the pluripotent state establishes memory but can be re-established by switching back to the primed state of hiPSCs. These findings suggest that iPSC memory is likely governed by mechanisms that go beyond incomplete methylation or modified histone status that allow for unique marking and requiring transcriptional plasticity after apparent erasure. This may form the basis for the distinguishing feature of mouse versus human iPSCs in the context of somatic memory, where serial passage of hiPSCs is unable to remove memory. Lentivirus preparation and induction of hiPSCs Plasmids pSIN-EF2-OCT4-Pur, pSIN-EF2-SOX2-Pur, pSIN-EF2-Nanog-Pur, pSIN-EF2-LIN28-Pur, pSIN4-EF2-O2S, pSIN4-EF2-N2L and pSIN-CMV-K2M were gifts from James A. Thomson (University of Madison-Wisconsin). These vectors were transfected with second-generation packaging plasmids (psPAX2 and pMD2.G) in a 293FT cell line. Viral supernatant were collected 48 h after transfection, concentrated with ultracentrifugation and titred with HeLa cells [2] . Human dermal Fibs (ScienCell) or human CB cells from healthy donors (two independent Fibs donors and three CB samples) were transduced with concentrated lentiviral vectors in the presence of 8 μg ml −1 polybrene (Millipore). Informed consent was obtained from all sample donors in accordance with Research Ethics Board-approved protocols at McMaster University and the London Health Science Centre. CD34 + CB cells, used for hCB-iPSCs generation, were isolated by immunomagnetic separation. Transduced cells were maintained on irradiated feeder mouse embryonic fibroblasts (MEFs) in Dulbecco’s modified Eagle’s medium (DMEM)/F12 (Gibco) supplemented with 20% Knockout Serum Replacement (Gibco), 100 μM β-mercaptoethanol, 100 μM nonessential amino acid (Gibco), 1 mM L -glutamine (Gibco) and 10 ng ml −1 basic fibroblast growth factor (bFGF). hiPSCs were examined for the expression of pluripotent markers including OCT4, cell surface stage-specific antigen 3 (SSEA3), SSEA4 and TRA1-60. Specific primer sets were used to detect pluripotent genes and are listed in Supplementary Table 1 . Human ESCs and iPSCs cultures The hESC line and Fibs-hiPSCs were cultured on Matrigel (BD Biosciences) in MEF-conditioned medium (MEF-CM) supplemented with 8 ng ml −1 bFGF (Invitrogen) as previously described [28] . Fib hiPSCs and umbilical CB hiPSCs were cultured on irradiated feeder MEFs in DMEM/F12 (Gibco) with 20% Knockout Serum Replacement (Gibco), 100 μM β-mercaptoethanol, 100 μM nonessential amino acid (Gibco), 1 mM L -glutamine (Gibco) and 10 ng ml −1 bFGF. Cells were fed with fresh medium daily and confluent cultures were mechanically passed using 1 mg ml −1 collagenase IV (Invitrogen). Naive hiPSCs were derived based on previous reports [23] , [24] , [25] and maintained with 1 μM MEK inhibitor PD0325901, 3 μM GSK3 inhibitor CHIR99021 and 10 ng ml −1 LIF. Teratoma assay The McMaster University Animal Care Council approved all procedures and protocols. Undifferentiated hiPSCs (1.0 × 10 6 cells per mouse) were mechanically collected, resuspended in PBS and then injected intratesticularly into male non-obese diabetic/severe combined immunodeficient (NOD/SCID) [28] . Mice were killed 8 weeks after initial injection. Teratomas were collected, embedded in paraffin, sectioned followed by deparaffinization in xylene and processing through a graded series of alcohol concentrations. Samples were stained with haematoxylin and eosin followed by dehydration and xylene treatment. Images were acquired using ScanScope CS digital slide scanner (Aperio, CA, USA). hEB formation and hematopoietic differentiation hiPSCs cultured on irradiated MEFs (iMEFs) were depleted of iMEFs, split and seeded onto Matrigel-coated plates, and then cultured for 7 days with MEF-CM supplemented with 8 ng ml −1 bFGF (Invitrogen). To generate hematopoietic cells from hiPSCs, we generated hEBs [29] . Confluent undifferentiated hiPSCs were treated with 200 U ml −1 collagenase IV for 5–10 min and then transferred to 6- or 12-well ultralow attachment plates (Corning). Clumps of hiPSCs were incubated overnight to allow hEB formation in the hEB-differentiation medium supplemented with hematopoietic growth factors as follows: 50 ng ml −1 granulocyte colony-stimulating factor (Amgen Inc., Thousand Oaks, CA, USA), 300 ng ml −1 stem cell factor (SCF; Amgen), 10 ng ml −1 interleukin-3 (R&D systems, Minneapolis, MN, USA), 10 ng ml −1 interleukin-6 (R&D systems), 25 ng ml −1 BMP4 (R&D systems) and 300 ng ml −1 Flt-3 ligand (Flt-3L: R&D systems). hEBs were cultured for 7–15 days and the medium was changed every 3 days. Colony-forming unit assay CFU assay was performed by plating single-cell suspensions from hEBs into methylcellulose H4434 (Stem Cell Technologies, Vancouver, BC, Canada) [13] . hEBs were dissociated with collagenase B and cell-dissociation buffer and then filtered through a 40-μm cell strainer. Dissociated hEBs were counted and plated into methylcellulose H4434 in 24- or 12-well ultralow attachment plates. For characterization of hematopoietic colony-forming capability from haemangioblasts, 1 × 10 3 cells were purified from blast cultures at day 6 and resuspended in 20 μl of Stemline II medium and mixed well with 0.5 ml of methylcellulose H4436 (Stem Cell Technologies) as previously assayed [19] . After 14 days, differential colony counts were performed based on morphology. Generation of haemangioblasts Haemangioblasts were generated as previously described [19] . Briefly, hEBs were cultured in hEB-differentiation medium (Stemline II (Sigma) supplemented with 50 ng ml −1 BMP4 and vascular endothelial growth factor (R&D Systems)) for 48 h, and then replaced with Stemline II medium containing 50 ng ml −1 BMP4, 50 ng ml −1 vascular endothelial growth factor and 20 ng ml −1 bFGF. After 24 h, hEBs were collected, dissociated into single-cell suspension and resuspended in Stemline II medium and then plated in blast growth medium (BGM) for up to 6 days. Differentiation into erythroid cells Erythroid differentiation and expansion was carried out as previously described [21] . Briefly, haemangioblasts at day 6 were collected and cultured in BGM medium supplied with 3 U ml −1 erythropoietin and cultured for 5–7 days until confluence. To further expand, cells were collected and replated in BGM medium with 3 U ml −1 erythropoietin. For further differentiation and maturation, expanded cells were cultured with BGM medium mixed with StemPro-34 SCF medium at 1:1 ratio. SCF (100 ng ml −1 ) and 3 units ml −1 erythropoietin were added to media. β-globin protein expression was detected after 6 days in culture. Plating in BGM medium after hEB dissociation was denoted as day 0 of erythroid culture. Differentiation into endothelial cells Purified haemangioblasts were plated on fibronectin-coated plate with EGM-2 medium (Lonza) as previously described [19] . Endothelial cells were cultured for 30 days. Expression of the endothelial-specific marker PECAM (BD Biosciences) on differentiated endothelial cells was confirmed by immunofluorescence staining. Low-density lipoprotein (LDL) uptake was evaluated by culturing the cells in the presence of 10 μg ml −1 Alexa Fluor 594 Ac-LDL (Invitrogen) for 8 h. The expression of endothelial markers and intracellular LDL staining was examined using fluorescence microscopy. Neurosphere generation and neural differentiation For neural differentiation, the hiPSCs, cultured on iMEFs, were depleted of feeders, seeded onto Matrigel-coated plates and then cultured for 7 days with MEF-CM supplemented with 8 ng ml −1 bFGF and then EBs were generated with EB medium without cytokines as previously described [22] . After 4 days in suspension culture, EBs were plated onto poly- L -lysine/laminin-coated plates (BD Biosciences) in neural differentiation medium composed of DMEM/F12 with B27 (Gibco) and N2 (Gibco) supplements, 25 ng ml −1 EGF (R&D Systems), 2.5 ng ml −1 IGF (R&D Systems), 25 ng ml −1 platelet-derived growth factor (PDGF)-AA (R&D Systems) and 8 ng ml −1 bFGF. After 5 days under this condition, EBs were collected for fluorescence-activated cell sorting analysis. Neurosphere expansion and subsequent differentiation were carried out as previously described [11] , [12] . Briefly, the hiPSCs, cultured on iMEFs, were depleted of feeders, seeded onto Matrigel-coated plates and then cultured for 7 days with MEF-CM supplemented with 8 ng ml −1 bFGF. hEBs were generated by suspension culture with neural-proliferation media (DMEM/F12 supplemented with 1 × N2, 1 × B27, 20 ng ml −1 EGF and 20 ng ml −1 FGF-2). hEBs were cultured for 7 days with a media change every other day. For neurosphere formation and expansion, hEBs were collected and dissociated into single cells with Accutase (Sigma). Dissociated single cells were plated into low-attachment 6-well plates (2 × 10 5 cells per well) in neural-proliferation media to facilitate neurosphere formation over 7 days. Media was changed every 3 days. After 7 days, neurospheres were collected, dissociated into single cells and counted. To quantify neurosphere generation capacity of hiPSCs, minimal numbers of cells (1,000) at the end of expansion cycles were cultured with neural proliferating media and neurosphere were counted. Neural precursors were analysed for the neural stem cell marker nestin (R&D Systems) and the neural precursor marker A2B5 (R&D Systems) by flow cytometry. To differentiate neural precursors along the neuronal lineage, cells were plated onto poly- L -lysine/laminin-coated plates (BD Biosciences) grown in DMEM F12 supplemented with 1 × N2, 1 × B27, all-trans Retinoic acid (Sigma) at 2 μM and forskolin (Sigma) at 5 μM. To induce astrocytic differentiation, neural precursors were cultured in DMEM/F12 supplemented with 1 × N2, 1 × B27 and 5% fetal bovine serum. Oligodendrocyte differentiation was induced by culturing cells in DMEM/F12, 1% N2, 1% B27 and IGF-1 (200 ng ml −1 ). In all conditions, cells were allowed to differentiate for 1 week. In vitro hepatocytic differentiation For hepatocyte differentiation, the hiPSCs seeded onto Matrigel-coated plates, and then cultured for 5 days with MEF-CM supplemented with 8 ng ml −1 bFGF and then replaced with RPMI supplemented with 1 × B27, 100 ng ml −1 activin A, 10 ng ml −1 hepatocyte growth factor and 1 μM CHIR99021 (GSK3 inhibitor) for 3 days of endoderm formation as previously described [30] . Then cell medium was replaced with knockout-DMEM with 20% knockout-SR, 1 mM L -glutamine, 1% nonessential amino acids, 0.1 mM β-mercaptoethanol and 1% dimethyl sulfoxide for 4 days. For maturation, the cells were cultured in Iscove's modified Dulbecco's medium (IMDM) containing 20 ng ml −1 oncostatin M, 0.5 μM dexamethasone and 50 mg ml −1 ITS premix. Flow cytometry analysis Single-cell suspensions were stained using the following antibodies: CD31-PE (1:100) (BD Pharmingen), CD34-PE or -FITC (1:100) (Miltenyi Biotech, Bergisch Gladbach, Germany), CD45-APC (1:100) (Miltenyi Biotech), SSEA-1 (1:100), SSEA-3 (1:100), SSEA-4 (1:100) (Developmental Studies Hybridoma Bank), TRA1-60-Alexa Fluor 647 (1:500), TRA1-85-APC (1:500), OCT4 (1:200) (BD Biosciences), A2B5 (1:100), Nestin (1:500), Oligodendrocyte Marker O4 (1:200), Neuron-specific beta-III Tubulin (1:200) (R&D Systems), GFAP (1:200) (Sigma) and Haemoglobin β-PerCP (1:500) (Santa Cruz). Unconjugated antibodies were visualized with appropriated Fluorochrome-conjugated secondary antibody. Fluorescence-activated cell sorting analysis was performed on a FACSCalibur cytometer (Becton Dickinson Immunocytometry Systems) and analysed using FlowJo software (Tree Star Inc). Immunocytochemistry Immunostaining was performed as previously described [13] . Briefly, cells were fixed in 4% paraformaldehyde and stained with appropriate antibodies. If permeation was needed, cells were treated with 0.1% saponin (BD Biosciences) prior to staining. Appropriate primary and fluorochrome-conjugated secondary antibodies were used. Cells were then counterstained with Hoechst 33342 (Invitrogen) or mounted with Vectashield Mounting Medium containing 4',6-diamidino-2-phenylindole (DAPI) (Vector Labs). The following antibodies were used: SSEA-1 (1:100), SSEA-3 (1:100), SSEA-4 (1:100), OCT4 (1:200), TRA-1-60-Alexa Fluor 488 (1:100) (BD Biosciences), GFAP (1:200), Oligodendrocyte Marker O4 (1:200), Neuron-specific beta-III Tubulin (1:200) and Haemoglobin β (1:100) (Santa Cruz). Alexa Fluor 488-conjugated secondary antibody was used for SSEA-1, SSEA-3, SSEA-4 and Oligodendrocyte Marker O4, and Alexa Fluor 555-conjugated secondary antibody was used for OCT4, GFAP, Neuron-specific beta-III Tubulin and Haemoglobin β. Quantitative RT-PCR Total RNA was extracted from cells using the RNeasy kit (Qiagen). Complementary DNA (cDNA) was made with 1 μg of total RNA using the first-strand cDNA synthesis kit (Invitrogen) and subsequent quantitative real-time PCR (Q-PCR) was carried out in triplicate, using SYBR Green reverse transcriptase (RT)-PCR reagents (Applied Biosystems) on an Mx3000P Q-PCR System according to the manufacturer’s instructions (Stratagene). Amplifications were performed using the following conditions: 95°C for 10 min, followed by 40 cycles of 95 °C for 15 s and 60 °C for 1 min. All data were normalized to glyceraldehyde 3-phosphate dehydrogenase (GAPDH). Primer sequences used were shown in Supplementary Table 1 . Affymetrix analysis Total RNA for microarrays was isolated using the RNA isolation kit (Invitrogen). RNA was hybridized to Affymetrix Human Gene 1.0 ST arrays (London Regional Genomics Centre, ON, Canada). Array data were normalized using the robust multichip averaging method and baseline transformed to the median of all samples (GeneSpring 12.0, Agilent Technologies). Hierarchical clustering using Pearson distance metric and centroid linkage rule was done on normalized expression values of all entities. Unsupervised GSEA was done on normalized expression values of all entities between hCB- and hFib-iPSCs samples using GSEA software v2.07 (Broad Institute). Curated (C2v3.0) and gene ontology (C5v3.0) gene sets from Molecular Signatures Database (MSigDB) were used. Gene sets were filtered based on permutation on gene sets with n =1,000 permutations. Enrichment plots were generate on statistically significant relevant functional gene sets: mesoderem, ectoderm, endoderm, heart development (Gene Ontology), neuronal lineage (KEGG, Reactome, and previously reported data [31] ), hepatocytic lineage [32] and hematopoietic lineage [15] , [16] from published data. Chromatin immunoprecipitation assays Chromatin immunoprecipitation (ChIP) experiments were performed as previously described [22] . For each condition, 1 × 10 6 cells (Fib-derived or CB-derived iPS) were collected and cross-linked using 1% formaldehyde. Chromatin was fragmented by sonication in buffer containing 1% NP-40 to obtain fragments of ~250 bp length. Sonicated DNA was subjected to immunoprecipitation using anti-trimethyl H3K4 (07-473, Millipore), anti-trimethyl H3K27 (17-622 ChIPAb+, Millipore) and anti-rabbit IgG (17-622 ChIPAb+, Millipore) antibodies. Immunoprecipitated DNA was further reverse cross-linked, purified and subjected to Q-PCR analysis to detect MixL1 , Brachyury (T), Pax6 and NF68 promoter fragments. Sequence enrichment was calculated relative to input signal. Specific primers used to amplify each promoter sequence were described in Supplementary Table 2 . Methylated DNA-pulldown analysis Fractionation of methylated double-stranded DNA was performed using the MethylMiner methylated DNA enrichment kit according to manufacturer’s recommendations (ME10025, Invitrogen). Briefly, 1 × 10 6 Fib-derived or CB-derived iPS cells were collected and genomic DNA was extracted using the DNeasy Blood and Tissue kit (#69504, Qiagen). Fragmentation of genomic DNA was performed by sonication (~250 bp length) and methylated DNA portions were pulled down based on their interaction with the methyl-CpG-binding domain (MBD) of human MBD2 protein immobilized on beads. Purified fragments were analysed by Q-PCR to assess for the enrichment of MixL1 , Brachyury (T), Pax6 and NF68 promoter sections, relative to input material. Specific primers used to amplify each promoter sequence were described in Supplementary Table 2 . Statistical analysis All results were expressed as means±s.e.m. and generated from at least three independent experiments. Statistical significance was determined using the Student’s t -test and results were considered significant or highly significant when P <0.05 or P <0.01, respectively. How to cite this article: Lee, J.-H. et al. Somatic transcriptome priming gates lineage-specific differentiation potential of human-induced pluripotent stem cell states. Nat. Commun. 5:5605 doi: 10.1038/ncomms6605 (2014). Accession codes: All array data have been uploaded to Gene Expression Omnibus ( http://www.ncbi.nlm.nih.gov/geo/ ) under accession codes GSE62066 .